γ-Glutamylcysteine detoxifies reactive oxygen species by acting as glutathione peroxidase-1 cofactor Reactive oxygen species regulate redox-signaling processes, but in excess they can cause cell damage, hence underlying the aetiology of several neurological diseases. Through its ability to down modulate reactive oxygen species, glutathione is considered an essential thiol-antioxidant derivative, yet under certain circumstances it is dispensable for cell growth and redox control. Here we show, by directing the biosynthesis of γ-glutamylcysteine—the immediate glutathione precursor—to mitochondria, that it efficiently detoxifies hydrogen peroxide and superoxide anion, regardless of cellular glutathione concentrations. Knocking down glutathione peroxidase-1 drastically increases superoxide anion in cells synthesizing mitochondrial γ-glutamylcysteine. In vitro , γ-glutamylcysteine is as efficient as glutathione in disposing of hydrogen peroxide by glutathione peroxidase-1. In primary neurons, endogenously synthesized γ-glutamylcysteine fully prevents apoptotic death in several neurotoxic paradigms and, in an in vivo mouse model of neurodegeneration, γ-glutamylcysteine protects against neuronal loss and motor impairment. Thus, γ-glutamylcysteine takes over the antioxidant and neuroprotective functions of glutathione by acting as glutathione peroxidase-1 cofactor. Mitochondria are both producers and targets of reactive oxygen species (ROS). A well-balanced equilibrium between mitochondrial ROS production and their elimination is critical for the control of redox-mediated cell signalling processes [1] . By disposing ROS, glutathione (γ-glutamylcysteinylglycine, GSH) is thought to be the main small thiol-antioxidant derivative [2] , [3] . GSH is synthesized exclusively in the cytosol in two consecutive ATP-requiring steps, the first of which, and rate limiting, being γ-glutamylcysteine formation by glutamate-cysteine ligase (GCL); glutathione synthetase (GSS) then forms the tripeptide by linking glycine to γ-glutamylcysteine [2] , [3] . It is well documented that pharmacological inhibition of GCL activity [4] or knockdown of the catalytic GCL subunit [5] increases ROS abundance, which mediates cellular damage; GCL genetic deletion is embryonically lethal [6] , [7] . Interestingly, GSH is dispensable for the cell growth of Saccharomyces cerevisiae genetically deleted of GSS [8] . In addition, it has been recently demonstrated that, in S. cerevisiase devoid of GSS, GSH is essential for iron–sulfur cluster assembly, but not for thiol-redox control [9] . Both in yeast [8] and in human fibroblasts [10] , genetic GSS deletion results in γ-glutamylcysteine accumulation; thus the antioxidant function of GSH might be adopted by γ-glutamylcysteine. Here we tested whether—and if so, how—γ-glutamylcysteine detoxifies hydrogen peroxide (H 2 O 2 ) and superoxide anion (O 2 ·– ) under intact, physiological GSH concentrations. To do so, GCL was directed to mitochondria, as this organelle cannot further transform γ-glutamylcysteine into GSH due to the absence of GSS [11] . We found that both mitochondrial-targeted newly synthesized, and endogenous γ-glutamylcysteine, efficiently dispose H 2 O 2 by acting as glutathione peroxidase-1 cofactor. These results indicate that γ-glutamylcysteine is an important player in cellular redox control. Targeting functional GCL to mitochondria decreases ROS To direct γ-glutamylcysteine synthesis to mitochondria, the full-length complementary DNA encoding the catalytic GCL subunit was fused with the mitochondrial-targeting signal of ornithine transcarbamylase. When expressed in HEK293T cells, this construct ( mito GCL) yielded a GCL protein that was confined to mitochondria and absent in the cytosol, as revealed by western blotting after cellular fractionation ( Fig. 1a ) and confocal microscopy ( Fig. 1b ). In contrast, expression of untagged GCL was exclusively present in the cytosol ( Fig. 1a,b ). Whole-cell extracts expressing mito GCL revealed a super-shifted anti-GCL (1:1,000) band that was not present in the untagged GCL-expressing cells or in the mito GCL-transfected mitochondria ( Fig. 1c ), suggesting that only the mitochondrial-targeting epitope-processed form of the protein was present in the mitochondrial fraction. 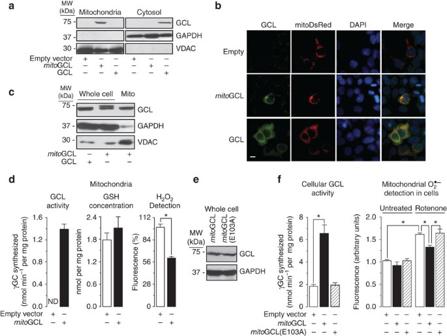Figure 1: Targeting glutamate-cysteine ligase to mitochondria decreases ROS. (a) Expression of GCL fused with the mitochondrial epitope of ornithine transcarbamylase (mitoGCL) in HEK293T cells shows localization in the mitochondrial, not in the cytosolic fraction, as judged by western blotting. Native (untagged) GCL is exclusively expressed in cytosol. (b) Confocal images show co-localization ofmitoGCL with the mitochondrial marker mitoDsRed, whereas native GCL showed typical cytosolic diffused pattern. Cells nuclei were stained with 4,6-diamidino-2-phenylindole (DAPI). Scale bar, 10 μm. (c) Whole extracts of cells expressingmitoGCL shows both native and mitochondrial-tagged GCL, as judged by the loss of the super-shifted band in the mitochondrial fraction. (d)mitoGCL is functional, as judged by the presence of GCL activity (synthesis of γ-glutamylcysteine, γGC) in the mitochondrial fraction (left panel); mitochondrial GSH concentration was unaltered bymitoGCL expression, whereas the rate of H2O2production(AmplexRed), after treatment with 10 μM rotenone, significantly decreased (right panel). (e) Expression of the wild-type (mitoGCL) and the E103A inactive mutant form ofmitoGCL showed identical protein abundance. (f) The E103A mutantmitoGCL form is inactive (left panel), as judged by the lack of γGC formation in transfected cells; rotenone (1 μM per 4 h) induced an increase in mitochondrial superoxide anion (O2·–) abundance, as revealed by MitoSox fluorescence detection followed by flow cytometry; this increase was partially prevented by the wild-type, but not by the E103A mutant inactivemitoGCL form (right panel). Mitochondrial enrichment was assessed by VDAC (Voltage Dependent Anion Channel) immunoblotting. The cytosolic enzyme GAPDH (glyceraldehyde-3-phosphate dehydrogenase) was used to assess equal loading in immunoblots. ND, not detected; *P<0.05 (analysis of variance;n=3 independent experiments). All data are expressed as mean±S.E.M±. Figure 1: Targeting glutamate-cysteine ligase to mitochondria decreases ROS. ( a ) Expression of GCL fused with the mitochondrial epitope of ornithine transcarbamylase ( mito GCL) in HEK293T cells shows localization in the mitochondrial, not in the cytosolic fraction, as judged by western blotting. Native (untagged) GCL is exclusively expressed in cytosol. ( b ) Confocal images show co-localization of mito GCL with the mitochondrial marker mitoDsRed, whereas native GCL showed typical cytosolic diffused pattern. Cells nuclei were stained with 4,6-diamidino-2-phenylindole (DAPI). Scale bar, 10 μm. ( c ) Whole extracts of cells expressing mito GCL shows both native and mitochondrial-tagged GCL, as judged by the loss of the super-shifted band in the mitochondrial fraction. ( d ) mito GCL is functional, as judged by the presence of GCL activity (synthesis of γ-glutamylcysteine, γGC) in the mitochondrial fraction (left panel); mitochondrial GSH concentration was unaltered by mito GCL expression, whereas the rate of H 2 O 2 production(AmplexRed), after treatment with 10 μM rotenone, significantly decreased (right panel). ( e ) Expression of the wild-type ( mito GCL) and the E103A inactive mutant form of mito GCL showed identical protein abundance. ( f ) The E103A mutant mito GCL form is inactive (left panel), as judged by the lack of γGC formation in transfected cells; rotenone (1 μM per 4 h) induced an increase in mitochondrial superoxide anion (O 2 ·– ) abundance, as revealed by MitoSox fluorescence detection followed by flow cytometry; this increase was partially prevented by the wild-type, but not by the E103A mutant inactive mito GCL form (right panel). Mitochondrial enrichment was assessed by VDAC (Voltage Dependent Anion Channel) immunoblotting. The cytosolic enzyme GAPDH (glyceraldehyde-3-phosphate dehydrogenase) was used to assess equal loading in immunoblots. ND, not detected; * P <0.05 (analysis of variance; n =3 independent experiments). All data are expressed as mean±S.E.M±. Full size image Then, we assessed whether expressed mito GCL yielded functional GCL within mitochondria. As shown in Fig. 1d (left panel), GCL activity was undetectable in mitochondria isolated from control cells, but present in mito GCL-transfected cells. Furthermore, neither mitochondrial ( Fig. 1d , middle panel) nor cytosolic ( Supplementary Fig. S1a ) GSH concentrations changed by mito GCL expression. Interestingly, H 2 O 2 detection was significantly diminished by mito GCL expression, as measured both in mitochondria ( Fig. 1d , right panel) and in intact cells ( Supplementary Fig. S1b,c ). Expression of mito GCL prevented the conversion of GSH to its oxidized form (GSSG) caused by rotenone ( Supplementary Fig. S1d ). To confirm that GCL activity wholly accounted for ROS down-modulation, we expressed ( Fig. 1e ) a E103A mutant [12] , inactive ( Fig. 1f , left panel) form of mito GCL. We found that rotenone-induced mitochondrial O 2 ·– was significantly decreased by wild-type mito GCL, but not by the E103A inactive form ( Fig. 1f , right panel). These data confirm that γ-glutamylcysteine is required for the observed antioxidant function. γ-Glutamylcysteine is a GPx1 cofactor that detoxifies H 2 O 2 To decipher how γ-glutamylcysteine detoxified ROS but otherwise avoiding the influence of cytosolic GCL, we expressed a silent mutant mito GCL form ( mito GCL (mut)) refractory to the action of a small hairpin RNA against GCL (shGCL) [5] , in HEK293T cells ( Fig. 2a ). Knocking down GCL markedly reduced total cellular GSH in both mito GCL and mito GCL (mut) transfected cells ( Supplementary Fig. S1e ). GCL knockdown was insufficient to trigger a significant increase in mitochondrial O 2 ·– , but this was strongly potentiated by rotenone and rescued by mito GCL (mut; Fig. 2b ). Thus, in unstressed HEK293T cells, γ-glutamylcysteine may not contribute to the basal O 2 ·– regulation that can occur in primary neurons, in which we previously reported a significant increase in O 2 ·– by shGCL [13] . It therefore appears that the impact of γ-glutamylcysteine as a physiological redox regulator differs among cell types. Next, we knocked down GSS ( Fig. 2c ), which resulted in endogenous γ-glutamylcysteine accumulation and GSH decrease ( Supplementary Table S1 ). We found that GSS knockdown abolished the increase in rotenone-induced O 2 ·– , both in the absence ( Supplementary Fig. S1f ) and in the presence of mito GCL ( Fig. 2d ). 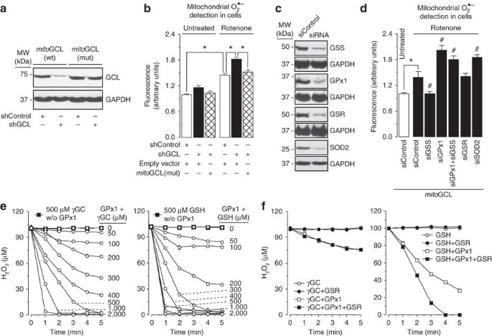Figure 2: γ-Glutamylcysteine is a GPx1 cofactor detoxifying mitochondrial H2O2. (a) Expression of an shRNA against GCL (shGCL) in HEK293T cells efficiently knockdowns wild-typemitoGCL, but not a mutant form ofmitoGCL (mitoGCL (mut)) that is refractory to shGCL. (b) Treatment of cells with rotenone (1 μM; 4 h) increased mitochondrial O2·–, as revealed by MitoSox fluorescence; this was further enhanced by GCL silencing (shGCL), and rescued bymitoGCL (mut) expression; GCL silencing in the absence of rotenone did not significantly modify mitochondrial O2·–in HEK293T cells (c) Western blots showing the efficacy of siRNA duplexes, used at 100 nM for 3 days in HEK293T cells, against glutathione synthetase (GSS), glutathione peroxidase-1 (GPx1), glutathione reductase (GSR) and superoxide dismutase-2 (SOD2); control siRNA (siControl) was an siRNA against luciferase. GAPDH (glyceraldehyde-3-phosphate dehydrogenase) was used as loading control. (d) Rotenone (1 μM; 4 h) increased mitochondrial O2·–, as judged by MitoSox fluorescence, inmitoGCL-expressing cells; this effect was abolished by GSS silencing and enhanced by GPx1 knockdown; silencing GSS did not rescue the increase in O2·–caused by GPx1 knockdown; GSR silencing did not alter, and SOD2 silencing enhanced rotenone-induced ROS. (e) γ-Glutamylcysteine (γGC) or GSH dose-dependently disposed H2O2in vitro, but the presence of GPx1 (0.5 U ml−1) in the incubation medium was necessary for H2O2disposal, as judged by the lack of effect of 500 μM γGC or GSH in the absence of GPx1 (w/o GPx1). (f) H2O2disposal by GPx1 was not potentiated by the presence of GSR (0.5 U ml−1) in the incubation medium when γGC (200 μM) was used (left panel); however, the presence of GSH (200 μM) potentiated GPx1-mediated H2O2disposal (right panel). *P<0.05;#P<0.05 versus siControl (mitoGCL; analysis of variance;n=3 independent experiments);in vitroassays (eandf) were performed in sextuplicate. All data are expressed as mean±S.E.M. Figure 2: γ-Glutamylcysteine is a GPx1 cofactor detoxifying mitochondrial H 2 O 2 . ( a ) Expression of an shRNA against GCL (shGCL) in HEK293T cells efficiently knockdowns wild-type mito GCL, but not a mutant form of mito GCL ( mito GCL (mut)) that is refractory to shGCL. ( b ) Treatment of cells with rotenone (1 μM; 4 h) increased mitochondrial O 2 ·– , as revealed by MitoSox fluorescence; this was further enhanced by GCL silencing (shGCL), and rescued by mito GCL (mut) expression; GCL silencing in the absence of rotenone did not significantly modify mitochondrial O 2 ·– in HEK293T cells ( c ) Western blots showing the efficacy of siRNA duplexes, used at 100 nM for 3 days in HEK293T cells, against glutathione synthetase (GSS), glutathione peroxidase-1 (GPx1), glutathione reductase (GSR) and superoxide dismutase-2 (SOD2); control siRNA (siControl) was an siRNA against luciferase. GAPDH (glyceraldehyde-3-phosphate dehydrogenase) was used as loading control. ( d ) Rotenone (1 μM; 4 h) increased mitochondrial O 2 ·– , as judged by MitoSox fluorescence, in mito GCL-expressing cells; this effect was abolished by GSS silencing and enhanced by GPx1 knockdown; silencing GSS did not rescue the increase in O 2 ·– caused by GPx1 knockdown; GSR silencing did not alter, and SOD2 silencing enhanced rotenone-induced ROS. ( e ) γ-Glutamylcysteine (γGC) or GSH dose-dependently disposed H 2 O 2 in vitro , but the presence of GPx1 (0.5 U ml −1 ) in the incubation medium was necessary for H 2 O 2 disposal, as judged by the lack of effect of 500 μM γGC or GSH in the absence of GPx1 (w/o GPx1). ( f ) H 2 O 2 disposal by GPx1 was not potentiated by the presence of GSR (0.5 U ml −1 ) in the incubation medium when γGC (200 μM) was used (left panel); however, the presence of GSH (200 μM) potentiated GPx1-mediated H 2 O 2 disposal (right panel). * P <0.05; # P <0.05 versus siControl ( mito GCL; analysis of variance; n =3 independent experiments); in vitro assays ( e and f ) were performed in sextuplicate. All data are expressed as mean±S.E.M. Full size image We then sought to elucidate if γ-glutamylcysteine served as a glutathione peroxidase cofactor. As glutathione peroxidase-1 (GPx1) largely accounts for mitochondrial H 2 O 2 detoxification [14] , we knocked down it ( Fig. 2c ), which resulted in a significant enhancement of rotenone-induced O 2 ·– ( Fig. 2d ). Furthermore, GSS knockdown was unable to decrease O 2 ·– levels during GPx1 silencing ( Fig. 2d ). The oxidized form of γ-glutamylcysteine was undetectable in cultured cells ( Supplementary Table S1 ), but it was present in all tissues analysed in vivo (brain, liver and kidney; Supplementary Table S2 ). Knocking down glutathione reductase (GSR) failed to enhance rotenone-induced O 2 ·– ( Fig. 2d ). To disregard a direct interaction of γ-glutamylcysteine with O 2 ·– , we silenced the mitochondrial isoform of superoxide dismutase (SOD2; Fig. 2c ), which enhanced rotenone-induced O 2 ·– ( Fig. 2d ). The ability of either γ-glutamylcysteine or its cognate cofactor, GSH, to dispose H 2 O 2 in vitro was then assessed in the absence or presence of purified GPx1. As shown in Fig. 2e , γ-glutamylcysteine and GSH were unable to detoxify H 2 O 2 , unless GPx1 was present; γ-glutamylcysteine dose-dependently accelerated GPx1-mediated H 2 O 2 disposal at a similar efficiency to that by GSH, at least at low concentrations of the thiols ( Fig. 2e ). GSR failed to improve the GPx1-dependent ability of γ-glutamylcysteine, but not that of GSH, at disposing H 2 O 2 ( Fig. 2f ). We also tested the ability of γ-glutamylcysteine to induce protein modification, which was found to be well below that of GSH ( Supplementary Table S3 ). mito GCL decreases ROS in neurons and is neuroprotective Neurons are particularly vulnerable against excess ROS, hence requiring continuous supply and regeneration of GSH for survival [15] . We therefore investigated the possible efficacy of γ-glutamylcysteine at detoxifying ROS in (patho) physiologically relevant neuronal death models. Glutamate treatment increased mitochondrial O 2 ·– in rat primary neurons ( Fig. 3a ; Supplementary Fig. S2a ), an effect that was abolished by the N -methyl- D -aspartate receptor antagonist [16] , MK801 ( Supplementary Fig. S2b ). Expression of mito GCL in neurons was sufficient to decrease basal mitochondrial O 2 ·– ( Fig. 3a ), which contrasts with the lack of effect in HEK293T cells ( Fig. 1f ). The different response of these cells to mito GCL expression is likely due to the above-mentioned vulnerability of neurons to oxidative stress [15] versus the resistance of HEK293T cells ( Fig. 2b ). Furthermore, mito GCL, but not its inactive E103A mutant form, prevented the increase in mitochondrial O 2 ·– induced by glutamate-receptor stimulation ( Fig. 3a ). GPx1—but not GSS or GSR—knockdown ( Supplementary Fig. S2c ) significantly enhanced O 2 ·– ( Fig. 3b ), despite neurons expressed mito GCL, indicating that GPx1 use of γ-glutamylcysteine is essential for γ-glutamylcysteine-mediated O 2 ·– detoxification in this model of excitotoxicity. Glutamate triggered an increase in the proportion of neurons with active caspase-3 ( Fig. 3c ) and with annexin V + /7-AAD − staining ( Fig. 3d ), indicating an intrinsic (mitochondrial) mode of apoptotic death; this was prevented by antagonizing the N -methyl- D -aspartate receptors ( Supplementary Fig. S2d,e ). Notably, mito GCL largely—but not fully—prevented the rise in the percentage of neurons with the apoptotic phenotype ( Fig. 3c,d ). In addition, mito GCL abolished O 2 ·– enhancement triggered by other mitochondrial ROS-inducing agents [17] , [18] , such as rotenone, antimycin and 3-nitropropionic acid (3NP; Fig. 3e ). 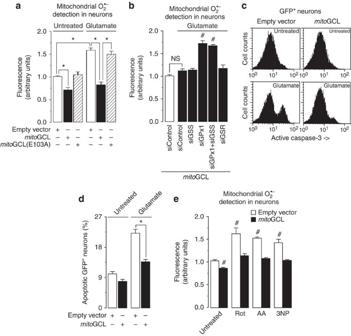Figure 3:mitoGCL down-modulates mitochondrial superoxide in primary neurons. (a) Transfection of rat primary neurons withmitoGCL, but not with its inactive form (mitoGCL (E103A)), significantly decreased basal levels of mitochondrial O2·–, as quantified by MitoSox fluorescence in the transfected neurons (identified by GFP+fluorescence);mitoGCL—but notmitoGCL (mut)—fully prevented glutamate (100 μM per 5 min)-induced mitochondrial O2·–, as quantified 24 h after glutamate treatment, by MitoSox fluorescence. (b) Silencing glutathione peroxidase-1 (siGPx1), but not glutathione synthetase (siGSS) or glutathione reductase (siGSR), significantly enhanced glutamate (100 μM per 5 min)-mediated mitochondrial O2·–, as judged by MitoSox fluorescence 24 h after treatment, inmitoGCL-expressing neurons; such enhancement was not affected by GSS co-silencing. (c) Expression ofmitoGCL rescued the increase, observed after 24 h, in active caspase-3 in GFP+-neurons triggered by glutamate (100 μM per 5 min), as assessed by flow cytometry. (d)mitoGCL expression prevented neuronal apoptotic death, as revealed by annexin V+/7-AAD−neurons 24 h after glutamate treatment (100 μM per 5 min). (e)mitoGCL expression prevented the increase in mitochondrial O2·–(as assessed by MitoSox fluorescence) caused by incubation of neurons with rotenone (Rot, 10 μM), antimycin A (AA, 10 μM) or 3-nitropropionic acid (3NP, 2 mM) for 15 min. NS, not significant; *P<0.05;#P<0.05 versus untreated (analysis of variance;n=3 independent culture preparations). All data are expressed as mean±S.E.M. Figure 3: mito GCL down-modulates mitochondrial superoxide in primary neurons. ( a ) Transfection of rat primary neurons with mito GCL, but not with its inactive form ( mito GCL (E103A)), significantly decreased basal levels of mitochondrial O 2 ·– , as quantified by MitoSox fluorescence in the transfected neurons (identified by GFP + fluorescence); mito GCL—but not mito GCL (mut)—fully prevented glutamate (100 μM per 5 min)-induced mitochondrial O 2 ·– , as quantified 24 h after glutamate treatment, by MitoSox fluorescence. ( b ) Silencing glutathione peroxidase-1 (siGPx1), but not glutathione synthetase (siGSS) or glutathione reductase (siGSR), significantly enhanced glutamate (100 μM per 5 min)-mediated mitochondrial O 2 ·– , as judged by MitoSox fluorescence 24 h after treatment, in mito GCL-expressing neurons; such enhancement was not affected by GSS co-silencing. ( c ) Expression of mito GCL rescued the increase, observed after 24 h, in active caspase-3 in GFP + -neurons triggered by glutamate (100 μM per 5 min), as assessed by flow cytometry. ( d ) mito GCL expression prevented neuronal apoptotic death, as revealed by annexin V + /7-AAD − neurons 24 h after glutamate treatment (100 μM per 5 min). ( e ) mito GCL expression prevented the increase in mitochondrial O 2 ·– (as assessed by MitoSox fluorescence) caused by incubation of neurons with rotenone (Rot, 10 μM), antimycin A (AA, 10 μM) or 3-nitropropionic acid (3NP, 2 mM) for 15 min. NS, not significant; * P <0.05; # P <0.05 versus untreated (analysis of variance; n =3 independent culture preparations). All data are expressed as mean±S.E.M. Full size image mito GCL exerts neuroprotection in vivo To confirm that γ-glutamylcysteine exerted neuroprotection in vivo , lentiviral particles expressing wild-type or inactive (E103A) mito GCL were stereotaxically injected into the striatum of adult mice. After 3 days, striatal GCL activity was significantly higher in mice injected with mito GCL than in those injected with inactive mito GCL (E103A), whereas striatal GSH concentrations remained unchanged ( Fig. 4a ). After 3 days of lentiviral injections, mice were intraperitoneally injected with 3NP (seven doses of 50 mg kg −1 , twice daily), a well-described model of neurodegeneration [18] . Indeed, we observed that 3NP treatment induced a significant increase in neuronal apoptotic death in the striatum, as judged by TdT-mediated dUTP nick end labelling assay, in the mice pre-injected with inactive mito GCL (E103A), but not in those pre-injected with wild-type mito GCL ( Fig. 4b,c ). Notably, there was a significant loss of striatal neurons in the mice pre-injected with the inactive mito GCL (E103A), but not in those pre-injected with the wild-type mito GCL ( Fig. 4d ; Supplementary Fig. S2f ). Mice treated with vehicle instead of 3NP showed no neuronal loss, regardless of the isoform of mito GCL (wild type or inactive) pre-injected ( Fig. 4d ; Supplementary Fig. S2f ). To evaluate behavioural function, these mice were tested for motor coordination and balance. As shown in Fig. 4e , 3NP treatment induced a progressive motor impairment in the mice that were pre-injected with the inactive mito GCL (E103A), but not in those pre-injected with the wild-type mito GCL; mice treated with vehicle instead of 3NP showed no motor impairment, regardless of the isoform of mito GCL (wild type or inactive) pre-injected ( Fig. 4e ). 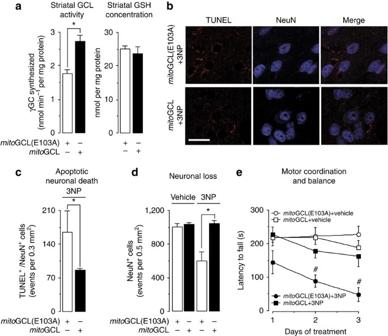Figure 4:mitoGCL exerts neuroprotectionin vivo. (a) Lentiviral particles expressing wild-type or inactive (E103A)mitoGCL were stereotaxically injected (5×106p.f.u. per 3 μl at 0.25 μl min−1) into the striatum of adult mice. After 3 days, striatal GCL activity was significantly higher in mice injected withmitoGCL than in those injected with inactivemitoGCL (E103A), whereas striatal GSH concentrations remained unchanged. (b) Confocal images of striatal sections showing neuronal apoptotic death. After 3 days of lentiviral particles injections, 3NP was intraperitoneally injected (seven doses of 50 mg kg−1, twice daily), which induced a significant increase in neuronal apoptotic death (TUNEL+/Neu+cells) in the striatum, in the mice pre-injected with inactivemitoGCL (E103A), but not in those pre-injected with wild-typemitoGCL; scale bar, 20 μm. (c) This panel shows the quantitative data ofb. (d) After 3 days of lentiviral particles injections, 3NP was intraperitoneally injected, which induced, 3 days later, a significant loss of striatal NeuN+neurons only in the mice that received inactivemitoGCL (E103A), but not in those that received wild-typemitoGCL; mice treated with vehicle instead of 3NP showed no neuronal loss regardless of the isoform ofmitoGCL (wild type or inactive) lentiviral particles injected; the quantitative analysis is shown. (e) After 3 days of lentiviral particles injections, 3NP was intraperitoneally injected, which induced, 3 days later, a progressive motor impairment (rotarod test) in mice pre-injected with inactivemitoGCL (E103A), but not with wild-typemitoGCL; mice treated with vehicle, instead of 3NP, showed no neuronal loss, regardless of the isoform ofmitoGCL (wild type or inactive) pre-injected. *P<0.05;#P<0.05 versus all conditions on each day (Student'st-test for (a,c);n=3 mice; analysis of variance for (d,e);n=6–8 mice). TUNEL, TdT-mediated dUTP nick end labelling. All data are expressed as mean±S.E.M. Figure 4: mito GCL exerts neuroprotection in vivo . ( a ) Lentiviral particles expressing wild-type or inactive (E103A) mito GCL were stereotaxically injected (5×10 6 p.f.u. per 3 μl at 0.25 μl min −1 ) into the striatum of adult mice. After 3 days, striatal GCL activity was significantly higher in mice injected with mito GCL than in those injected with inactive mito GCL (E103A), whereas striatal GSH concentrations remained unchanged. ( b ) Confocal images of striatal sections showing neuronal apoptotic death. After 3 days of lentiviral particles injections, 3NP was intraperitoneally injected (seven doses of 50 mg kg −1 , twice daily), which induced a significant increase in neuronal apoptotic death (TUNEL + /Neu + cells) in the striatum, in the mice pre-injected with inactive mito GCL (E103A), but not in those pre-injected with wild-type mito GCL; scale bar, 20 μm. ( c ) This panel shows the quantitative data of b . ( d ) After 3 days of lentiviral particles injections, 3NP was intraperitoneally injected, which induced, 3 days later, a significant loss of striatal NeuN + neurons only in the mice that received inactive mito GCL (E103A), but not in those that received wild-type mito GCL; mice treated with vehicle instead of 3NP showed no neuronal loss regardless of the isoform of mito GCL (wild type or inactive) lentiviral particles injected; the quantitative analysis is shown. ( e ) After 3 days of lentiviral particles injections, 3NP was intraperitoneally injected, which induced, 3 days later, a progressive motor impairment (rotarod test) in mice pre-injected with inactive mito GCL (E103A), but not with wild-type mito GCL; mice treated with vehicle, instead of 3NP, showed no neuronal loss, regardless of the isoform of mito GCL (wild type or inactive) pre-injected. * P <0.05; # P <0.05 versus all conditions on each day (Student's t -test for ( a , c ); n =3 mice; analysis of variance for ( d , e ); n =6–8 mice). TUNEL, TdT-mediated dUTP nick end labelling. All data are expressed as mean±S.E.M. Full size image Here we show that γ-glutamylcysteine is a thiol-redox regulator that efficiently detoxifies mitochondrial ROS. This was evidenced by confining γ-glutamylcysteine synthesis to mitochondria, which were unable to convert the newly synthesized γ-glutamylcysteine into GSH due to the lack of mitochondrial GSS [11] . Thus, down-modulation of mitochondrial ROS by γ-glutamylcysteine took place under physiological GSH concentrations. Furthermore, the robust antioxidant protection observed in intact GSS knockdown cells corroborates such a role by endogenous γ-glutamylcysteine. Notably, impairing γ-glutamylcysteine biosynthesis in the cytosol, but not in mitochondria, still allowed γ-glutamylcysteine to efficiently detoxify ROS. Together, these results indicate that the antioxidant action of γ-glutamylcysteine takes place regardless of GSH concentrations, thus cannot simply rely on its ability to replenish GSH, as it can be seen in other paradigms [19] . Our results also reveal that GPx1 is an essential component in the detoxifying function of γ-glutamylcysteine. Furthermore, the occurrence of an oxidized form of γ-glutamylcysteine in all tissues analysed, in vivo , strongly suggests the notion of a γ-glutamylcysteine redox cycle. However, knocking down GSR—presumably required for an eventual regeneration of reduced γ-glutamylcysteine from its oxidized form—failed to enhance O 2 ·– . The biochemical pathway responsible for the reduction of γ-glutamylcysteine from its oxidized form therefore remains to be elucidated. On the other hand, a putative function of γ-glutamylcysteine as direct superoxide anion scavenger is disregarded, as SOD2 knockdown could not further enhance rotenone-induced O 2 ·– . Our data obtained by knocking down GPx1, both in the human HEK293T cells and in rat neurons, together with the in vitro experiments, strongly suggest that endogenous γ-glutamylcysteine is a GPx1 cofactor for H 2 O 2 detoxification. It cannot be ruled out that γ-glutamylcysteine could also act as a cofactor for other isoforms of the glutathione peroxidase family; however, GPx1 largely accounts for most mitochondrial H 2 O 2 detoxification [14] , suggesting a major role for this isoform. Moreover, previous studies have shown that GPx1 can accept, albeit at a much lower efficiency, a range of thiol-derivatives besides GSH as the electron donor [20] . The essential cysteinyl-sulfhydryl and glutamyl-carboxylic groups for GPx1 active site interaction and catalysis [14] are both preserved in γ-glutamylcysteine, indicating the structural feasibility for this function. Due to its very low ability to synthesize and regenerate GSH, the brain is one of the most vulnerable tissues to excess ROS [15] , [21] . In Parkinson's disease, there is an ~60% reduction in GSH concentration in the substantia nigra of presymptomatic patients [22] , suggesting GSH deficiency as one of the earliest biochemical signs of this disorder. Moreover, signs of excess ROS are associated with the pathophysiology of other neurodegenerative diseases, such as Alzheimer's, or disorders affecting motor functional disturbances such as Amyotrophic Lateral Sclerosis or Huntington's disease [23] . At the light of our data, GPx1 is essential for γ-glutamylcysteine-mediated ROS detoxification and neuroprotection against different insults triggering neurodegeneration in primary neurons. Furthermore, we also show neuroprotection and motor improvement in an in vivo mouse model of neurodegeneration [18] . Thus, targeting γ-glutamylcysteine to neuronal mitochondria represents an improvement over the protection activity of neighbouring astrocytes [24] , [25] . In conclusion, our results demonstrate that γ-glutamylcysteine is a thiol-redox regulator that efficiently detoxifies mitochondrial ROS through GPx1. In the presence of γ-glutamylcysteine taking an antioxidant function, GSH stops from being oxidized; moreover, the ability of γ-glutamylcysteine to induce protein modification is well below that of GSH. Thus, when γ-glutamylcysteine takes the antioxidant functions, GSH utilization may be preserved for iron–sulfur cluster assembly and protein thiol-redox modifications, as recently reported [9] . How the antioxidant role of γ-glutamylcysteine is regulated under (patho) physiological conditions now needs to be deciphered. In this context, it should be noted that, besides GCL, alternative pathways can account for intracellular γ-glutamylcysteine [2] , [3] . For instance, γ-glutamyltransferase forms γ-glutamylcysteine at the extracellular side of the plasma membrane and then is taken up by the cells through the glutamyl-amino acid transporter [2] . It would be interesting to investigate if increased γ-glutamylcysteine could explain the drug resistance observed in tumours associated with γ-glutamyltransferase overexpression [26] . In addition, whether GSH deficiency is the prime mode of the pro-oxidant actions of the GCL/GSS/glutamyl-amino acid transporter inhibitor, L -buthionine sulfoximine [4] needs to be revisited. Finally, our results, showing neuroprotection by mitochondrial-targeted γ-glutamylcysteine biosynthesis, supports the oxidative hypothesis of neurodegeneration [27] . Although classical antioxidant drugs failed in clinical trials against neurodegenerative disorders [28] , mito GCL, by acting as a persistent antioxidant source for mitochondria, may represent a new gene therapy strategy to improve the transient efficacy of the formers. Plasmids and lentivirus construction To tag the catalytic subunit of human GCL with a mitochondrial-targeting epitope, the 5′-end of the full-length (2,023 bp) cDNA-encoding GCL (GenBank accession number NM_012815 ) was fused with a cDNA fragment encoding the first 32 amino acids of human ornithine transcarbamylase (GenBank accession number NM_000531 ). The forward and reverse oligonucleotides of this fragment were, respectively, 5′- GATCT ATGCTGTTTAATCTGAGGATCCTGTTAAACAATGCAGCTTTTAGAAATGGTCACA ACTTCATGGTTCGAAATTTTCGGTGTGGACAACCACTACAAG-3′ and 5′- AATTC TTGTAGTGGTTGTCCACACCGAAAATTTCGAACCATGAAGTTGTGACCATTTCTA AAAGCTGCATTGTTTAACAGGATCCTCAGATTAAACAGCATA-3′ ( Bgl II and Eco RI sites underlined; Thermo Scientific, Offenbach, Germany). The fused cDNA construct ( mito GCL) was inserted in pIRES2-EGFP (Invitrogen) vector and sequence-verified; mito GCL was then subcloned into pcDNA3.1 + (Invitrogen) and pIRES2-DsRed2 (Clontech Laboratories Inc., Palo Alto, CA, USA) with Nhe I/ Sma I or Nhe I/ Xma I restriction enzymes, respectively. For lentiviral particles production, the full-length cDNA-encoding mito GCL, or its mutant inactive E103A form, was first digested with Eco 47III /Sma I to generate blunt ends, and then subcloned in the Pme I site of pWPI lentiviral vector (Didier Trono laboratory, Lausanne, Switzerland). Recombinant lentiviruses were generated following a standard protocol [29] . Viral titters were determined by incubation of 3T3 cells with increasing dilutions of lentivirus in the presence of 8 μg ml −1 polybrene (Millipore), followed by green fluorescent protein (GFP) quantification by flow cytometry. Lentiviral particles were re-suspended to a final concentration of 1.7×10 6 plaque formation untis (p.f.u.) per μl. To direct GCL expression to the cytosol, we used non-tagged GCL. To knockdown GCL by small hairpin RNA (shRNA), a vector-based shRNA approach using the targeting sequence 5′-GAAGGAGGCTACTTCTATA-3′, as we described [5] , was used. The firefly luciferase-targeted oligonucleotide 5′-CTGACGCGGAATACTTCGA-3′ was used as control [30] . The forward and reverse 64-nt-long oligonucleotides were annealed and inserted into the Bgl II/ Hin dIII sites of pSuper-neo/GFP vector (OligoEngine, Seattle, WA). These constructions concomitantly express 19-bp, 9-nucleotide stem-loop shRNAs with GFP, thus allowing the identification of transfected cells by fluorescence microscopy and flow cytometry. Small interfering RNA construction Using previously reported rational criteria [31] , [32] , we designed the following target sequences to get gene expression-specific knockdown by short interfering RNA (siRNA). For GSS: 5′-AGGAAATTGCTGTGGTTTA-3′ (nucleotides 856–874 for human NM_000178) and 5′-AGAGAAGGAAAGAAACATA-3′ (nucleotides 713–731 for rat NM_012962). For GSR: 5′-AGACGAATTCCAGAATACC-3′ (nucleotides 1211–1229 for human NM_000637) and 5′-GGACCTGAGTTTAAACAAA-3′ (nucleotides 1154–1172 for rat NM_053906). For glutathione peroxidase-1 (GPx1): 5′-CGCCAAGAACGAAGAGATT-3′ (nucleotides 338–356 for both human, NM_00581, and rat, NM_030826.3). SOD2 or MnSOD: 5′-GGGAGTTGCTGGAAGCCAT-3′ (nucleotides 381–399 for both human, NM_000636, and rat, NM_017051). In all cases, a siRNA against luciferase (5′-CTGACGCGGAATACTTCGATT-3′) was used as control. siRNAs were purchased from Dharmacon (Abgene, Thermo Fisher, Epsom, UK). Site-directed mutagenesis Mutant forms of mito GCL refractory to the shRNA against GCL ( mito GCLmut) or catalytically inactive mito GCL ( mito GCL (E103A)) were generated using the site-directed mutagenesis QuikChange XL kit (Stratagene, La Jolla, CA, USA), followed by Dpn I digestion. The forward and reverse oligonucleotides of the sequence 5′-GAA A GA A GC C AC G TC A GT T -3′, carrying silent third-codon base point mutations (mutant nucleotides underlined) were used for mito GCLmut. To generate mito GCL (E103A), the forward and reverse oligonucleotides 5′-CAGAGTATGGGAGTTACATGATT GCA GGGACACCTGGCCAGCCGTACGGA-3′ (mutant nucleotides underlined) were used. Cell cultures Cortical neurons in primary culture were prepared from fetal Wistar rats (E16), seeded at 2.5×10 5 cells per cm 2 in 6- or 12-well plates previously coated with poly- D -lysine (15 μg ml −1 ) in DMEM (Sigma, Madrid, Spain) supplemented with 10% (v/v) fetal calf serum (Roche Diagnostics, Heidelberg, Germany). Cells were incubated at 37 °C in a humidified 5% CO 2 -containing atmosphere. At 48 h after plating, the medium was replaced with DMEM supplemented with 5% horse serum (Sigma), 20 mM D -glucose and, on day 4, cytosine arabinoside (10 μM) to prevent non-neuronal proliferation [33] . Human embryonic kidney 293T (HEK293T) cells were maintained in DMEM supplemented with 10% (v/v) fetal calf serum. Cell transfections and treatments are specified in the Supplementary Methods . Cytosol was fractionated from mitochondria by differential centrifugation [34] . Primary antibodies for western blotting Immunoblotting was performed with rabbit polyclonal anti-GCL (1:1,000) [5] , rabbit polyclonal anti-GPX1 (1:1,000) (ab59546, Abcam, Cambridge, UK), rabbit polyclonal anti-GFP (1:1,000) (ab290, Abcam), mouse monoclonal anti-GSS (1:1,000) (Sc-166882, Santa Cruz Biotechnologies, Heidelberg, Germany), mouse monoclonal anti-GSR (Sc-133159, Santa Cruz Biotechnologies), mouse monoclonal anti-SOD2 (1:2,000) (ab16,956, Abcam), rabbit polyclonal anti-VDAC (1:1,000) (Calbiochem, Darmstadt, Germany) or mouse monoclonal anti-GAPDH (1:40,000) (glyceraldehyde-3-phosphate dehydrogenase; Ambion, Cambridge, UK) antibodies. VDAC and GAPDH were used as mitochondrial and cytosolic (or whole cell) loading controls, respectively. Determination of ROS Mitochondrial superoxide was detected using the fluorescent MitoSox probe (Invitrogen). Cells were incubated in Hank's buffer with 2 μM MitoSox-Red for 30 min at 37 °C in a 5% CO 2 atmosphere, washed with PBS and the fluorescence assessed by flow cytometry or fluorescence microscopy. We used the FL1, FL2 and FL3 channels of a FACScalibur flow cytometer (15 mW argon ion laser tuned at 488 nm; CellQuest software, Becton Dickinson Biosciences). Thresholds were adjusted by using non-stained and stained cells for MitoSOX fluorescence, and transfected and non-transfected cells for GFP fluorescence. For H 2 O 2 assessment in isolated mitochondria, 50 μg protein-aliquots of freshly obtained mitochondria were incubated with 100 μM AmplexRed probe (Invitrogen) in mitochondrial respiration buffer (125 mM KCl, 2 mM KH 2 PO 4 , 1 mM MgCl 2 , 0.5 mg ml −1 bovine serum albumin and 10 mM HEPES, pH 7.4) containing horseradish peroxidase (0.5 U ml −1 ). Luminescence was recorded for 45 min at 1 min intervals using a Fluoroskan Ascent FL (Thermo Scientific, Rockford, IL, USA) fluorimeter (excitation: 538 nm, emission: 604 nm), and the slopes were used for calculations. For H 2 O 2 assessment in whole cell, 1.5×10 4 cells were incubated in 100 μM AmplexRed in Krebs-Ringer Phosphate buffer (145 mM NaCl, 5.7 mM Na 2 PO 4 , 4.86 mM KCl, 0.54 mM CaCl 2 , 1.22 mM MgSO 4 and 5.5 mM glucose, pH 7.4), and the luminescence recorded as we did for mitochondria. Mitochondrial H 2 O 2 was also detected by fluorescence microscopy in seeded, intact cells following the green fluorescence emitted by cells transfected with pHyPer-dMito plasmid vector (Evrogen, Moscow, Russia), which express a mitochondrial-tagged H 2 O 2 -sensitive fluorescent probe. In vitro H 2 O 2 quantification was assessed as indicated in the Supplementary Methods . Determination of γ-glutamylcysteine level and GCL activity This was performed as described [35] . Cells were washed, colleted with 1 mM EDTA in PBS, pelleted (500 g for 5 min) and re-suspended in isolation medium (320 mM sucrose, 10 mM Tris–HCl, 1 mM EDTA, pH 7.4). Samples (whole cells or isolated mitochondria) were freeze-thawed three times, and the lysates filtered through 10-kDa molecular mass cutoff devices (Amicon, Millipore) at 12,000 g for 15 min at 4 °C. The retained protein fraction was immediately used for the determination of γ-glutamylcysteine concentration or assayed for GCL activity in 0.1 M Tris–HCl buffer containing 0.15 mM KCl, 20 mM MgCl 2 , 2 mM EDTA, 10 mM ATP, 10 mM L -cysteine, 40 mM L -glutamate and 220 μM acivicin, pH 8.2, at 37 °C for 15 min. The reaction was stopped by addition of ice-cold orthophosphoric acid (15 mM, final concentration), and the reaction product was immediately used for γ-glutamylcysteine determination. This was performed by high-pressure liquid chromatography using a LC-20A Shimadzu equipment (Shimadzu GmbH, Duisburg) with an interphase module (CBM-20A, Shimadzu GmbH) and electrochemical detection (ESA Biosciences, Inc., Chelmsford, MA), with the upstream electrode set at +100 mV (for compounds with low oxidation potential) and downstream electrode set between +100 and +650 mV (in +50 mV increments) for each injected standard to determine the optimum potential for detection. The samples were subjected to analysis with a Teknokroma MediterraneaSea 18 ODS column (4.6×250 mm, 5-μm particle size), using 15 mM orthophosphoric acid as the mobile phase [35] at a flow rate of 0.5 ml min −1 . An external standard of 2.5–10 μM γ-glutamylcysteine (Bachem, Germany) was used for the calculations. In preliminary experiments, we tested that γ-glutamylcysteine synthesis was linear with the incubation time at least up to 20 min. Glutathione and other thiols, disulphides, and protein disulphides formed with low-molecular-weight thiols were assayed by ultra performance liquid chromatography and mass spectrometric detection as described in Supplementary Methods . Protein determinations Cells or tissues were lysed in 0.1 M NaOH and used for the determination of protein concentrations, either by the method of Lowry et al ., as described [36] or by the BCA protein assay kit (Pierce), following the manufacturer's instructions. In both cases, bovine serum albumin was used as standard. Statistical analysis All measurements in cell culture were carried out, at least, in triplicate, and the results are expressed as the mean±s.e.m. values from at least three different culture preparations. For the rotarod experiments, we used six to eight animals per condition. Statistical analysis of the results was performed by one-way analysis of variance, followed by the least significant difference multiple range test or by the Student's t -test for comparisons between two groups of values. In all cases, P <0.05 was considered significant. Use of animals All animals used in this wok were obtained from the Animal Experimentation Unit of the University of Salamanca, in accordance with Spanish legislation (RD 1201/2005) under licence from the Spanish Ministry of Science and Innovation. Protocols were approved by the Bioethics Committee of the University of Salamanca. How to cite this article: Quintana-Cabrera, R. et al . γ-Glutamylcysteine detoxifies reactive oxygen species by acting as glutathione peroxidase-1 cofactor. Nat. Commun. 3:718 doi: 10.1038/ncomms1722 (2012).